Trans-regulation of oligodendrocyte myelination by neurons through small GTPase Arf6-regulated secretion of fibroblast growth factor-2 The small G protein ADP-ribosylation factor 6 (Arf6) plays important roles in a wide variety of membrane dynamics-based cellular events such as neurite outgrowth and spine formation in vitro . However, little is known about physiological function of Arf6 in vivo . Here we generate conditional knockout mice lacking Arf6 in neurons, oligodendrocytes, or both cell lineages, and unexpectedly find that Arf6 expression in neurons, but not in oligodendrocytes, is crucial for oligodendrocyte myelination in the hippocampal fimbria and the corpus callosum during development, and that this is through the regulation of secretion of fibroblast growth factor-2, a guidance factor for migration of oligodendrocyte precursor cells (OPCs). These results suggest that Arf6 in neurons plays an important role in OPC migration through regulation of FGF-2 secretion during neuronal development. Mammalian ADP-ribosylation factor (Arf) is a small GTPase cycling between an inactive GDP-bound and active GTP-bound form. Arf exists as the inactive GDP-bound form in the resting state of cells and becomes active by exchange of bound GDP for GTP in response to agonist stimulation of cells. The active state of Arf transduces signals to downstream effector molecules and thereafter hydrolyses GTP to GDP, to become the inactive state. These processes of guanine nucleotide exchange and GTP hydrolysis are regulated and accelerated by guanine nucleotide exchange factors and GTPase-activating proteins, respectively. The mammalian Arf family consists of six related gene products that are divided into three classes based on the sequence homology [1] . Class I includes Arf1, Arf2 and Arf3, class II Arf4 and Arf5, and class III Arf6. Arf classes I and II localize to the Golgi and endoplasmic reticulum, and primarily regulate vesicular trafficking between these organelles [2] , [3] . In contrast, Arf6 predominantly localizes to the plasma membrane and endosomal compartments, and through study of cell lines, has been proposed to regulate endocytosis of the plasma membrane, exocytosis, endosomal recycling and cytokinesis through re-organization of the actin cytoskeleton [4] . At a higher level and using similar approaches, Arf6 has been proposed to play an important role in axonal outgrowth and dendritic tree and spine formation [5] , [6] , suggesting that it should have critical neuronal functions in the central nervous system (CNS). However, in vivo roles for Arf6 in the nervous system have not yet been explored. We previously generated Arf6 knockout ( Arf6 -KO) mice to analyse Arf6 function in vivo , but full loss of Arf6 resulted in embryonic lethality [7] , preventing examination of the physiological function for Arf6 in the CNS. Here we examine this by generating and analysing conditional KO mice (CKO) lacking Arf6 in neurons, oligodendrocytes, or both cell lineages. We find that myelination of axons is impaired in the hippocampal fimbria (Fim) and the corpus callosum (CC) of neural stem cell (NSC)- and neuron-specific Arf6 -CKO mice. Furthermore, we find that Arf6 in neurons regulates migration of oligodendrocyte precursor cells (OPCs) through facilitating secretion of fibroblast growth factor-2 (FGF-2), a guidance factor for OPC migration. These results suggest that neuronal Arf6 plays an important role in directing OPC migration during neuronal development, thereby indirectly regulating oligodendrocyte myelination. Arf6 is required for axonal myelination in vivo We generated NSC-specific Arf6 conditional KO (NSC- Arf6 -CKO) mice that lacked expression of Arf6 in neurons and glia by mating Arf6 flox/flox mice with Nestin-Cre mice [8] (expression in other tissues, for example, the liver, remained at control levels; Supplementary Fig. 1a ). The NSC- Arf6 -CKO mice were viable as adult mice, although their brain weight was slightly but significantly reduced ( Supplementary Fig. 1b,c ). Histological inspection of the brain revealed that the size of the Fim and width of the CC in NSC- Arf6 -CKO mice were significantly reduced compared with control mice ( Fig. 1a–c ). As the Fim and CC primarily contain highly myelinated axons, myelination was analysed by luxol fast blue staining and was found to be profoundly decreased ( Fig. 1d ), which was confirmed by transmission electron microscopic (TEM) analysis ( Fig. 1e,f and Supplementary Fig. 2 ). In contrast, myelination in other regions of CNS, such as the fornix, cerebral peduncle and cerebellum, and the sciatic nerve of peripheral nervous system, was normal ( Supplementary Fig. 3 ), suggesting that the requirement of Arf6 for myelination is dependent on the neuronal subtype. 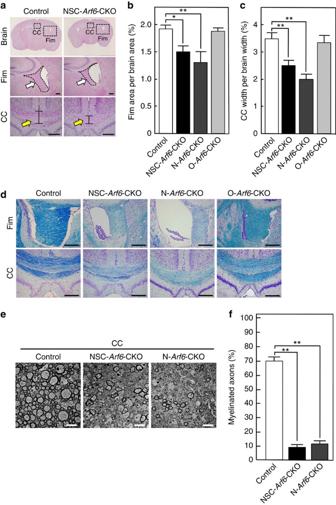Figure 1: Deletion ofArf6from neurons causes defective myelination in the Fim and CC during neuronal development. (a) Haematoxylin–eosin-stained sections of the brain of control and NSC-Arf6-CKO mice at P90. White arrows: Fim; yellow arrows: CC. Scale bar, 200 μm. (b,c) Area of Fim represented as percentage of brain area (b) and width of CC represented as percentage of brain width (c). (d) Luxol fast blue (LFB) staining of Fim and CC in control, NSC-Arf6-CKO, N-Arf6-CKO and O-Arf6-CKO mice at P90. Scale bar, 200 μm. (e) TEM of CC in control, NSC-Arf6-CKO and N-Arf6-CKO mice at P90. Scale bar, 2 μm. (f) Percentage of myelinated axons in CC of control, NSC-Arf6-CKO and N-Arf6-CKO mice at P90. Data shown are means±s.e.m. from three and four independent experiments for theb,candf, respectively. *P<0.05, **P<0.01, one-way analysis of variance with a Dunnett’s multiple comparison test. Figure 1: Deletion of Arf6 from neurons causes defective myelination in the Fim and CC during neuronal development. ( a ) Haematoxylin–eosin-stained sections of the brain of control and NSC- Arf6 -CKO mice at P90. White arrows: Fim; yellow arrows: CC. Scale bar, 200 μm. ( b , c ) Area of Fim represented as percentage of brain area ( b ) and width of CC represented as percentage of brain width ( c ). ( d ) Luxol fast blue (LFB) staining of Fim and CC in control, NSC- Arf6 -CKO, N- Arf6 -CKO and O- Arf6 -CKO mice at P90. Scale bar, 200 μm. ( e ) TEM of CC in control, NSC- Arf6 -CKO and N- Arf6 -CKO mice at P90. Scale bar, 2 μm. ( f ) Percentage of myelinated axons in CC of control, NSC- Arf6 -CKO and N- Arf6 -CKO mice at P90. Data shown are means±s.e.m. from three and four independent experiments for the b , c and f , respectively. * P <0.05, ** P <0.01, one-way analysis of variance with a Dunnett’s multiple comparison test. Full size image Arf6 in neurons is involved in axonal myelination To clarify in which cell type Arf6 expression is required for myelination, we generated neuron- and oligodendrocyte-specific Arf6 -CKO mice (referred to as N- Arf6 -CKO and O- Arf6 -CKO mice, respectively) by mating Arf6 flox/flox mice with Tau-Cre and 2′,3′-cyclic nucleotide 3′-phosphodiesterase (CNP)-Cre mice [9] , [10] , respectively. Unexpectedly, N- Arf6 -CKO mice but not O- Arf6 -CKO mice exhibited Fim and CC reductions in size ( Fig. 1b–d ) and fewer myelinated axons in the CC in adulthood ( Fig. 1d–f and Supplementary Fig. 4 ), similar to the NSC- Arf6 -CKO mice. As it has been reported that tau is expressed in oligodendrocyte lineage cells [11] , we examined whether Cre recombination occurs in oligodendrocytes of the Tau-Cre mice using LacZ reporter mice, but did not observe any such events ( Supplementary Fig. 5 ). These results suggest that Arf6 expression in neurons, but not in oligodendrocytes, is indispensable for myelination in the Fim and CC. Arf6 regulates axonal density and myelin thickness Quantitative TEM analysis of the CC revealed an increase in axonal density and a decrease in axon diameter in N- and NSC- Arf6 -CKO mice ( Fig. 2a,b ), which could be responsible for the decrease in the width of the CC. However, a small number of axons in N- and NSC- Arf6 -CKO mice in the Fim and CC remained myelinated ( Fig. 1e and Supplementary Fig. 2 ), which allowed us to examine myelin sheath thickness by analysing g-ratios [12] . The average g-ratio in the CC of the NSC- Arf6 -CKO mice was higher than that of control mice ( Fig. 2c ), demonstrating that the myelin sheath is thinner for those neurons that remained myelinated. 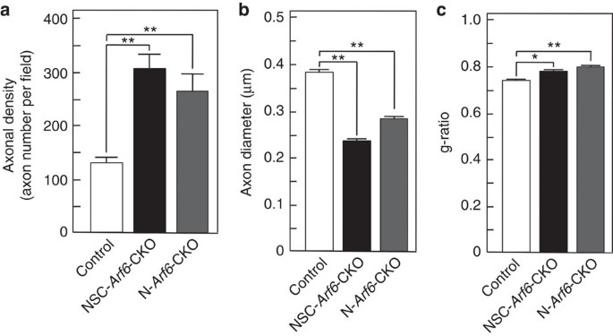Figure 2: Deletion of Arf6 from neurons increases axonal density and g-ratio, and decreases axon diameter in CC. The axonal density (a), the axon diameter (b) and g-ratio (c) in the CC of control, NSC-Arf6-CKO and N-Arf6-CKO mice were analysed using the TEM pictures shown inFig. 1e. Data shown are means±s.e.m. from four independent experiments. *P<0.05, **P<0.01, one-way analysis of variance with a Dunnett’s multiple comparison test. Figure 2: Deletion of Arf6 from neurons increases axonal density and g-ratio, and decreases axon diameter in CC. The axonal density ( a ), the axon diameter ( b ) and g-ratio ( c ) in the CC of control, NSC-Arf6-CKO and N-Arf6-CKO mice were analysed using the TEM pictures shown in Fig. 1e . Data shown are means±s.e.m. from four independent experiments. * P <0.05, ** P <0.01, one-way analysis of variance with a Dunnett’s multiple comparison test. Full size image Neuronal Arf6 is implicated in OPC migration Oligodendrocytes, the myelin-forming cells in CNS, originate from NSCs differentiating in the subventricular zone (SVZ). The OPCs differentiated from NSCs migrate to target sites such as the Fim and CC, and terminally differentiate there into oligodendrocytes that form myelin sheaths around nearby axons. Immunostaining for the OPC/oligodendrocyte-specific maker Olig2 in the Fim and CC revealed a decrease in the number of OPC/oligodendrocytes ( Fig. 3a,b and Supplementary Fig. 6 ) but no change in Olig2-negative cells ( Supplementary Fig. 7 ) in the N- and NSC- Arf6 -CKO mice. These results suggest that generation, migration and/or survival of OPCs/oligodendrocytes is impaired in these mice. The number of apoptotic cells in the Fim and CC was comparable between control and N- Arf6 -CKO mice ( Supplementary Fig. 8 ), and the generation of OPCs from NSCs in the SVZ was similarly normal in N- Arf6 -CKO mice at P5 ( Supplementary Fig. 9 ), as assessed by double-labelling of newly generated OPCs there with bromodeoxyuridine (BrdU) and the anti-Olig2 antibody. In contrast, the number of BrdU/Olig2 double-labelled OPCs in the Fim and CC in N- and NSC- Arf6 -CKO mice was significantly lower than that found in control animals ( Fig. 3c,d and Supplementary Fig. 10 ). These results, taken together, suggest that neuronal expression of Arf6 is involved in regulating OPC migration from the SVZ to these areas. 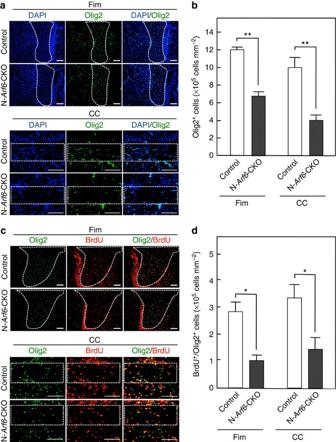Figure 3: Neuronally expressed ARF6 regulates migration of OPCs to the Fim and CC. (a) Fim and CC sections of control and N-Arf6-CKO mice at P14 were stained with anti-Olig2 antibody (green) and DAPI (blue). Scale bar, 100 μm. (b) The number of Olig2-positive cells inawas counted. (c) Fim and CC sections prepared from P14 control and N-Arf6-CKO mice injected with BrdU everyday during P1–10 were stained with anti-Olig2 antibody (green) and anti-BrdU antibody (red). Scale bar, 100 μm. (d) The number of BrdU/Olig2 double-positive cells in Fim and CC incwere counted. Areas of Fim and CC inaandcare outlined by dotted lines. Data shown are means±s.e.m. from three independent experiments. *P<0.05, **P<0.01, Student’st-test. Figure 3: Neuronally expressed ARF6 regulates migration of OPCs to the Fim and CC. ( a ) Fim and CC sections of control and N- Arf6 -CKO mice at P14 were stained with anti-Olig2 antibody (green) and DAPI (blue). Scale bar, 100 μm. ( b ) The number of Olig2-positive cells in a was counted. ( c ) Fim and CC sections prepared from P14 control and N- Arf6- CKO mice injected with BrdU everyday during P1–10 were stained with anti-Olig2 antibody (green) and anti-BrdU antibody (red). Scale bar, 100 μm. ( d ) The number of BrdU/Olig2 double-positive cells in Fim and CC in c were counted. Areas of Fim and CC in a and c are outlined by dotted lines. Data shown are means±s.e.m. from three independent experiments. * P <0.05, ** P <0.01, Student’s t -test. Full size image Arf6 regulates OPC migration by regulating FGF-2 secretion How might neuronal Arf6 regulate the migration of OPCs? OPC migration in vitro can be stimulated by guidance factors such as platelet-derived growth factor, FGF-2, Semaphorin 3A, epidermal growth factor, hepatocyte growth factor and glutamate [13] , [14] , which led us to speculate that the neuronal secretion of a critical guidance factor(s) might be Arf6 dependent. Supporting this hypothesis, OPC migration in vitro , which was elicited by co-culture with a hippocampal fragment in a Boyden chamber as shown in Supplementary Fig. 11 , was reduced by ~40% when the hippocampi were obtained from N- Arf6 -CKO mice ( Fig. 4a,b ). Thus, Arf6 appears to undertake a functional role in hippocampal neurons to regulate production and/or secretion of a guidance molecule(s) for OPC migration. 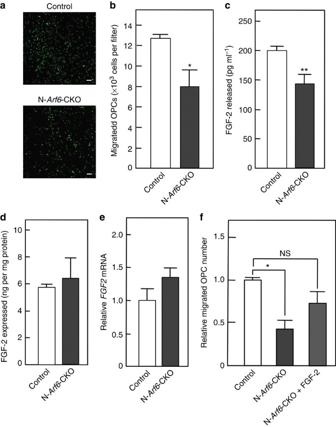Figure 4: Arf6 in hippocampal neurons regulates OPC migration through secretion of FGF-2. (a,b) OPCs that migrated to the lower surface of the membrane filter in Boyden chamber were stained for Olig2 (a) and the number of Olig2-positive cells counted (b). Scale bars, 200 μm. (c) FGF-2 secreted from hippocampi of control and N-Arf6-CKO mice into the culture medium. (d) FGF-2 protein levels in hippocampi of P7 control and N-Arf6-CKO mice. (e)FGF-2mRNA levels in hippocampi of P7 control and N-Arf6-CKO mice were measured. (f) N-Arf6-CKO hippocampi were cultured in the presence or absence of 0.1 ng ml−1FGF-2 in the lower Boyden chamber. OPCs that migrated to the lower surface of the membrane filter were counted. Data shown are means±s.e.m. from at least three independent experiments. *P<0.05, **P<0.01, n.s., not significant, Student’st-test for theb–eand one-way analysis of variance with a Dunnett’s multiple comparison test for thef. Figure 4: Arf6 in hippocampal neurons regulates OPC migration through secretion of FGF-2. ( a , b ) OPCs that migrated to the lower surface of the membrane filter in Boyden chamber were stained for Olig2 ( a ) and the number of Olig2-positive cells counted ( b ). Scale bars, 200 μm. ( c ) FGF-2 secreted from hippocampi of control and N- Arf6 -CKO mice into the culture medium. ( d ) FGF-2 protein levels in hippocampi of P7 control and N- Arf6 -CKO mice. ( e ) FGF-2 mRNA levels in hippocampi of P7 control and N- Arf6 -CKO mice were measured. ( f ) N- Arf6 -CKO hippocampi were cultured in the presence or absence of 0.1 ng ml −1 FGF-2 in the lower Boyden chamber. OPCs that migrated to the lower surface of the membrane filter were counted. Data shown are means±s.e.m. from at least three independent experiments. * P <0.05, ** P <0.01, n.s., not significant, Student’s t -test for the b – e and one-way analysis of variance with a Dunnett’s multiple comparison test for the f . Full size image An immediate candidate for the critical guidance factor is glutamate, as its secretion from purified synaptosomes requires Arf6 (ref. 15 ). However, glutamate release from cultured hippocampi was not affected by Arf6 ablation ( Supplementary Fig. 12 ). An alternative candidate was FGF-2, which is highly expressed in the hippocampus [16] . The secretion of FGF-2 from cultured N- Arf6 -CKO hippocampi was significantly decreased in comparison with control hippocampi ( Fig. 4c ), even though total protein expression and messenger RNA levels of FGF-2 were almost the same in the hippocampi from the control and N- Arf6 -CKO mice ( Fig. 4d,e ). Thus, Arf6 function in hippocampal neurons facilitates FGF-2 secretion, which suffices to explain the defect in OPC migration when Arf6 is absent. Supporting this hypothesis, addition of FGF-2 into the lower chamber with N- Arf6 -CKO hippocampal fragments restored OPC migration ( Fig. 4f ), indicating that the amount of FGF-2 released by N- Arf6 -CKO hippocampal fragments is rate limiting for OPC migration in culture . Collectively, the impairment of myelination at the Fim and CC of N- and NSC- Arf6 - CKO mice seems to be at least in part attributable to the suppression of FGF-2 secretion from neurons and the ensuing effects on OPC migration. The present study shows that deletion of the Arf6 gene from neurons but not from oligodendrocytes leads to defective myelination in the Fim and CC during neuronal development in vivo , suggesting that neuronal Arf6 is important for the development of myelination. In this study, we used the CNP promoter to drive Cre expression for generation of O- Arf6 -CKO mice, as CNP is detectable in OPCs at E11.5 to E12 and its expression is maintained in mature oligodendrocytes [17] . However, although this promoter-Cre system achieves essentially 100% targeted gene ablation in oligodendrocytes, CNP-Cre-mediated recombination is not 100% efficient for OPCs [18] . Accordingly, as some of the OPCs would still have expressed Arf6, we cannot totally exclude the possibility that Arf6 expression in OPCs as well as in neurons is involved in myelination, but we can fully exclude a role for Arf6 expression in oligodendrocytes. Another possibility is that the CNP-Cre promoter generates Cre activity in cell types other than oligodendrocytes at low frequencies, but this would not affect our conclusions. Most importantly, we can ascribe a role for neuronal Arf6 in the control of the myelination process, as the N- Arf6 -CKO but not the O- Arf6 -CKO mice generated in this study exhibited the myelination defect. To pursue the underlying mechanism, we analysed proliferation/differentiation of NSCs to OPCs/oligodendrocytes and migration of OPCs to the Fim and CC using Olig2/BrdU labelling. The results showed that the numbers of Olig2/BrdU-double-positive cells are unchanged in the SVZ but are reduced in the Fim and CC in the N- Arf6 -CKO mice. These results led to the conclusion that neuronal Arf6 plays an important role in OPC migration from the SVZ to the Fim and CC but not in NSC proliferation/differentiation, consistent with reports that OPCs differentiated from NSCs in the SVZ migrate to target areas in the postnatal brain [19] , [20] , [21] , [22] , [23] . However, it is still possible that proliferative NSCs in brain regions other than the SVZ differentiate into OPCs that migrate to the Fim and CC. Future studies that specifically label SVZ OPCs and trace their migration to the Fim and CC could be used to resolve this. OPC migration in vivo is elicited by guidance factors secreted by target tissues to which the OPCs migrate. We demonstrated in an in vitro system that Arf6 in the hippocampal tissue plays a crucial role in the secretion of the guidance factor FGF-2 that regulates OPC migration, consistent with reports showing that FGF-2 has a strong promoting effect on OPC migration [13] . To further extend the hypothesis that the Arf6-dependent FGF-2 secretion regulates OPC migration, in vivo experiments ablating FGF-2 receptors in OPCs or rescuing N- Arf6 -CKO mice through targeted provision of FGF-2 could be pursued. The myelin sheath has been reported to be thinner in mice lacking the FGF receptor [24] , indicating that FGF regulates myelin sheath formation. We found that Arf6 deletion from neurons decreased myelin sheath thickness, as evidenced by an increased g-ratio, accompanied by decreased secretion of FGF-2 as well. Our findings and hypothesis that Arf6 function in neurons is indirectly important for myelin sheath formation by facilitating the secretion of FGF-2 is thus consistent with this report [24] . FGF-2 is thought to be secreted through an unconventional pathway in which it translocates directly across the plasma membrane after being recruited to the plasma membrane by locally synthesized phosphatidylinositol 4,5-bisphosphate [25] . Considering the critical function of Arf6 in the activation of the phosphatidylinositol 4,5-bisphosphate-synthesizing enzyme phosphatidylinositol 4-phosphate 5-kinase (PIP5K) [26] , Arf6 could control FGF-2 secretion through PIP5K activation. Of three PIP5K isozymes, PIP5Kγ is specifically expressed in neurons [27] and its activation is dependent on its phosphorylation/dephosphorylation state: the phosphorylated form of PIP5Kγ present in resting cells is dephosphorylated on cellular stimulation to interact with AP-2 and talin, which then activate it [28] , [29] . However, it is unlikely that PIP5Kγ is involved in Arf6-dependent FGF-2 secretion, as its phosphorylation status was not changed by neuronal Arf6 ablation ( Supplementary Fig. 13 ). It would be of interest to test whether the other PIP5K isozymes, PIP5Kα and PIP5Kβ, might function as downstream effectors of Arf6 to facilitate FGF-2 secretion. Why was the defect in myelination caused by Arf6 deletion limited to the Fim and CC? Although it is well known that Arf6 regulates dense core vesicle secretion, membrane vesicle shedding and membrane trafficking along the axon [30] , [31] , [32] , all of which are important for neural secretion of biologically active substances [33] , [34] , [35] , neuronal subtypes found elsewhere than in the Fim and CC may secrete FGF-2 using an Arf6-independent mechanism(s). Alternatively, other guidance factors, such as platelet-derived growth factor, epidermal growth factor, hepatocyte growth factor and Semaphorin 3A [13] , may be secreted from distinct neuronal subtypes through mechanisms independent of Arf6. Mice Mouse experiments were conducted according to the Guideline for Proper Conduct of Animal Experiments, Science Council of Japan, and the protocol was approved by Animal Care and Use Committee, University of Tsukuba. Arf6 flox/flox mice (C57BL/6 background) were generated by a standard homologous recombination methods. Briefly, two lox P sites flanking exon 1 and 2 of Arf6 were introduced into genomic DNA covering the Arf6 gene of C57Bl/6J mice isolated from RPCI-23 BAC clone (Invitrogen) using standard restriction enzyme and PCR-based cloning techniques. A neomycin-resistance cassette ( neo ) flanked by FRT sites was also inserted between exon 2 and the second lox P site to prepare a targeting vector. The linearized targeting construct was electroporated into TT2 embryonic stem cells to obtain the recombinated Neo allele. Mice with floxed Arf6 allele were generated by mating mice with Neo allele with FLPe transgenic mice (a generous gift from Dr K. Araki, Kumamoto University). Nestin-Cre and CNP-Cre mice were provided by Drs Ryuichiro Kageyama (Kyoto University, Kyoto, Japan) and Klaus A. Nave (Max Planck Institute of Experimental Medicine, Göttingen, Germany), respectively [8] , [10] . Tau-Cre mice were generated as described previously [9] . NSC-, N- and O- Arf6 -CKO mice were generated by mating Arf6 flox/flox mice with Nestin-Cre, Tau-Cre and CNP-Cre mice, respectively. We used Arf6 flox/flox mice as a control in all experiments. To test whether Cre recombination occurs in Tau-Cre mice, they were crossed with Gt (ROSA) 26Sor lacZ reporter mice [9] . Analysis for Arf6 expression in tissues by western blotting The brain and liver dissected from mice were minced and homogenized on ice in buffer consisting of 20 mM Tris-HCl, pH 7.5, 1 mM EDTA and protease inhibitor cocktail (Nacalai Tesque), followed by the addition of SDS to make a final concentration of 1%. After sonication on ice and centrifugation at 1,000 g for 20 min at 4 °C, Arf6 in the supernatant was analysed by western blotting with anti-Arf6 antibody [36] as described previously [26] . Actin was also western blotted with anti-actin antibody (Sigma-Aldrich, MO, USA) as an internal standard. Arf6 and actin signals were visualized with the enhanced chemiluminescence detection reagent (Chemi-Lumi One, Nacalai Tesque) and the signal detected using LAS-4000Vmini (Fujifilm, Tokyo, Japan). Analysis of phosphorylation/dephosphorylation state of PIP5Kγ The lysates of the hippocampus and cerebral cortex dissected from mice were prepared as described in ‘Analysis for Arf6 expression in tissues by western blotting’. After separation on SDS–PAGE on 10% gels, PIP5Kγ was detected by western blotting with rabbit polyclonal anti-PIP5Kγ antibody, which was generated by immunization with a synthetic peptide corresponding to amino acids 622-635 of PIP5Kγ661 as described previously [26] . The lysates were treated with λ-PPase to dephospholylate PIP5Kγ and subjected to western blotting. Histological analysis and immunohistochemistry Mice were intracardially perfused with 4% paraformaldehyde (PFA) in PBS. Tissues were dissected and post-fixed in the same solution at 4 °C overnight. For haematoxylin and eosin staining and luxol fast blue staining, the post-fixed tissues were embedded in paraffin and sectioned at 5 μm using a microtome (REM-710, Yamato Kohki, Saitama, Japan) and stained using standard methods. For immunohistochemical staining, the post-fixed tissues were cryoprotected in 30% sucrose in PBS at 4 °C overnight, embedded in an optical coherence tomography compound (Sakura Finetek Japan, Tokyo, Japan) and sectioned at 10 μm using a cryostat (Leica Microsystems, Wetzlar, Germany). The sections in 10 mM EDTA (pH 8.0) were heated in a microwave oven, washed with PBS containing 0.1% Tween-20 and soaked in blocking solution (5% goat serum and 0.1% Tween-20 in PBS). After being incubated with rabbit antibody specific to Olig2 (1:200, Immuno-Biological Laboratories, Gunma, Japan) or cleaved caspase 3 (1:1,500; Cell Signaling), or mouse antibody to BrdU (1:1,000; Sigma-Aldrich) or lacZ (1:100; Promega) at 4 °C overnight, the sections were incubated with Alexa Fluor 488-conjugated goat antibody to rabbit or mouse IgG (1:1,000; Invitrogen, CA, USA) at room temperature for 2 h. In some experiment, the sections were counterstained with DAPI (4',6-diamidino-2-phenylindole; 4 ng ml −1 ; Molecular Probes, OR, USA) and imaged using a fluorescent microscope (Biozero BZ-8000, Keyence, Tokyo, Japan). Transmission electron microscopy TEM analysis was performed as previously described [37] with minor modifications. Briefly, mice were intracardially perfused with 2% PFA and 2% glutaraldehyde in 0.1 M cacodylate buffer, pH 7.4, and brain sections post-fixed with the same solution overnight at 4 °C. They were then treated with 1% OsO 4 in 0.1 M cacodylate buffer, pH 7.4, for 1 h, dehydrated in a graded series of ethanol and propylene oxide, and embedded in Epon. Semi-thin sections (0.5-μm-thick) of the Epon-embedded blocks were prepared by a Reichert-Jung ultramicrotome (Leica Microsystems, Wetzlar, Germany). Thin sections (90-nm-thick) were also prepared using a Reichert-Jung ultramicrotome and stained with a solution of uranyl acetate and lead citrate. The stained sections were observed by TEM on a JEM-1400 (JEOL, Tokyo, Japan) at 80 kV. Images were processed using a BZ-II Analyzer (Keyence). Percentage of myelinated axons and the g-ratio (diameter of an axon/diameter of an myelinated axon) were calculated by measuring 300–1,000 fibres. Analysis of differentiation in the SVZ Mice at P5 were intraperitoneally injected with 50 mg kg −1 of body weight of BrdU (Sigma-Aldrich). Two hours later, the mice were intracardially perfused with 4% PFA in PBS, the brain dissected and brain sections of 10-μm thickness prepared. The sections were stained with anti-Olig2 antibody and anti-BrdU antibody. BrdU/Olig2 double-positive and BrdU-positive cells in the SVZ were quantitated. Analysis of OPC migration from the SVZ to the Fim and CC Mice were daily injected with 50 mg kg −1 of body weight of BrdU from P1 to P10. At P14, the mice were perfused and the brains dissected as described above. Brain sections of 10 μm were prepared and immunostained for Olig2 and BrdU. BrdU/Olig2 double-positive cells in the Fim and CC were quantitated. Assay for in vitro migration of OPCs Migration of OPCs in vitro was assessed using a 24-well Boyden chamber (Corning Life Sciences, MA, USA). Forebrains dissected from P5 control mice were treated with 10 U ml −1 of papain and of DNase in DMEM medium (Nacalai Tesque, Kyoto, Japan) at 37 °C for 20 min. Dissociated cells were centrifuged at 1,000 g for 3 min, resuspended in DMEM supplemented with 10% fetal bovine serum, 100 U ml −1 penicillin and 100 μg ml −1 streptomycin, and seeded in the upper compartment of Boyden chambers at 5 × 10 5 cells per chamber. In the lower compartment of Boyden chambers, hippocampi dissected from P5 control and N- Arf6 -CKO mice were co-cultured in the same solution in the presence or absence of 0.1 ng ml −1 of FGF-2 at 37 °C under a humidified atmosphere containing 5% CO 2 . After 3 days, membrane filters were fixed with 4% PFA in PBS and stained with anti-Olig2 antibody. The number of Olig2-positive cells on the lower surface of the membrane filter was counted using the BZ-II Analyzer (Keyence). Quantification of glutamate and FGF2 release The amounts of glutamate and FGF2 secreted from hippocampi into the cultured medium were determined using the Glutamate Assay Kit (BioVision, CA, USA) and RayBio Mouse bFGF (FGF-2) ELISA Kit (RayBiotech, GA, USA), respectively, according to the manufacturer’s protocol. Hippocampi dissected from P5 control and N- Arf6 -CKO mice were cultured in 24-well dishes for 3 days as described in ‘Assay for in vitro migration of OPCs’. After culture media were collected and centrifuged by 1,000 g for 20 min, aliquots of 100 μl of the supernatants were used for analysis. Analysis of FGF2 expression in the hippocampus Hippocampal FGF2 protein and mRNA levels were determined using the RayBio Mouse bFGF (FGF-2) ELISA Kit and quantitative reverse transcription–PCR (qRT–PCR), respectively. For protein levels, dissected hippocampus from P7 mice were minced in ice-cold PBS, homogenized in 20 mM Tris-HCl, pH 7.5, 1 mM EDTA, and protease inhibitor cocktail, sonicated on ice, and centrifuged at 1,000 g for 20 min at 4 °C. An aliquot (100 μl) of the supernatant was analysed. For qRT–PCR, total RNA was extracted from P7 control and N-Arf6-CKO hippocampi using Trizol reagent (Invitrogen) following the manufacturer’s protocol. The RNA was treated with 2.5 U ml −1 RNase-Free DNase (Promega, WI, USA) in the presence of 20 U ml −1 RNAseOUT (Invitrogen) at 37 °C for 30 min to remove genomic DNA, followed by incubation at 95 °C for 15 min to inactivate the DNase. RNA (2 μg) was reverse-transcribed using SuperScript III Reverse Transcriptase (Invitrogen). qRT–PCR was performed using THUNDERBIRD SYBR qPCR Mix (Toyobo, Osaka, Japan) following the manufacturer’s protocol. Glyceraldehyde 3-phosphate dehydrogenase was used as an internal standard. The primer sequences used were as follows: FGF-2, 5′-CCAACCGGTACCTTGCTATGA-3′ and 5′-TTCGTTTCAGTGCCACATACCA-3′; glyceraldehyde 3-phosphate dehydrogenase, 5′-CATGGCCTTCCGTGTTCCTA-3′ and 5′-CCTGCTTCACCACCTTCTTGAT-3′. How to cite this article: Akiyama, M. et al. Trans -regulation of oligodendrocyte myelination by neurons through small GTPase Arf6-regulated secretion of fibroblast growth factor-2. Nat. Commun. 5:4744 doi: 10.1038/ncomms5744 (2014).